Tracing carbonate–silicate interaction during subduction using magnesium and oxygen isotopes Subduction of carbonates and carbonated eclogites into the mantle plays an important role in transporting carbon into deep Earth. However, to what degree isotopic exchanges occur between carbonate and silicate during subduction remains unclear. Here we report Mg and O isotopic compositions for ultrahigh pressure metamorphic marbles and enclosed carbonated eclogites from China. These marbles include both calcite- and dolomite-rich examples and display similar O but distinct Mg isotopic signatures to their protoliths. Their δ 26 Mg values vary from −2.508 to −0.531‰, and negatively correlate with MgO/CaO ratios, unforeseen in sedimentary carbonates. Carbonated eclogites have extremely heavy δ 18 O (up to +21.1‰) and light δ 26 Mg values (down to −1.928‰ in garnet and −0.980‰ in pyroxene) compared with their protoliths. These unique Mg–O isotopic characteristics reflect differential isotopic exchange between eclogites and carbonates during subduction, making coupled Mg and O isotopic studies potential tools for tracing deep carbon recycling. Deep carbon recycling plays a key role in the global carbon cycle by modulating the CO 2 budget of the Earth’s atmosphere over geologic timescales [1] , [2] . Among different subducted lithologies, carbonates and carbonated eclogites are of particular importance in transporting carbon from Earth’s surface into its interior [3] , [4] , [5] , [6] . As a subducting slab descends, some fractions of the carbon carried by carbonate minerals are liberated back at the surface via volcanism [7] ; however, most is delivered to great mantle depths together with silicates [8] , [9] . Carbonate–silicate interaction along the subduction pressure–temperature (P–T) paths is particularly important because it not only influences the long-term carbon flux in subduction zones [10] but also controls the isotopic systematics of coexisting carbonate and silicate that are ultimately recycled into the mantle. The latter in turn contributes fundamentally to the chemical and physical properties of the mantle [11] , [12] , [13] , for example, initiation of melting by lowering the mantle solidus, generation of alkalic magma in oceanic islands and carbonate metasomatism in cratonic mantle. Magnesium (Mg) and oxygen (O) are two essential elements closely associated with carbon in carbonate minerals. Their isotopic compositions differ greatly from normal mantle rocks, that is, unaltered oceanic basalts and lherzolites have δ 26 Mg of −0.25±0.07‰ (ref. 14 ) and δ 18 O of +5.5±0.2‰ (ref. 15 ), whereas sedimentary carbonates have extremely light δ 26 Mg (down to −6‰) [16] , [17] , [18] and heavy δ 18 O (up to +28‰) [19] , [20] . Thus, Mg–O isotopic systematics can provide insight into carbonate–silicate chemical interactions during the subduction of carbonates and carbonated eclogites. Here we present Mg, O, C and Nd isotopic data for a suite of ultrahigh pressure metamorphic (UHPM) marbles and enclosed carbonated eclogites from the Sulu orogen, east China. For comparison, we also report Mg isotopic data for Sinian sedimentary carbonates from the South China Block, and eclogites hosted in UHPM gneisses (termed as normal eclogites hereafter) from the Sulu orogen. Our results show that the carbonated eclogites have anomalously light δ 26 Mg and heavy δ 18 O as compared with the normal eclogites; moreover, UHPM marbles display negative correlation between δ 26 Mg and MgO/CaO. These Mg–O isotopic characteristics reflect differential isotopic exchange between the marble and enclosed eclogite during subduction, and provide important constraints on deep carbon recycling. Geologic setting and samples Triassic subduction of the South China Block beneath the North China Block resulted in the UHPM belts of Dabie and Sulu regions ( Supplementary Fig. 1a ) [21] . Eclogites are widespread as pods, discontinuous layers or blocks in gneisses, ultramafic massifs and marbles. Previous studies suggest that these eclogites were formed by UHP metamorphism of Neoproterozoic basaltic rocks during the Triassic subduction of the South China Block [21] , [22] , [23] , [24] . Diamond and coesite inclusions present in eclogites and their country rocks indicate that they were in situ subducted and exhumed with peak metamorphic temperatures of 700–880 °C and pressures up to 5.5 GPa (refs 25 , 26 , 27 ). The marble masses in the Rongcheng area crop out as large-scale discontinuous lenses with lengths of more than 2,000 m and are surrounded by orthogneisses containing layers or lenses of eclogites, amphibolites and serpentinized peridotites ( Supplementary Fig. 1b ). Samples studied here were collected from local marble quarries where many eclogites are present as centimetre- to metre-sized lenticular or spherical blocks in host marbles ( Supplementary Fig. 1c ). These marble-hosted eclogites are termed as carbonated eclogites hereafter. Field observation shows that the margins of carbonated eclogite blocks are invariably retrograded to amphibolites, while the cores are free of retrogression. 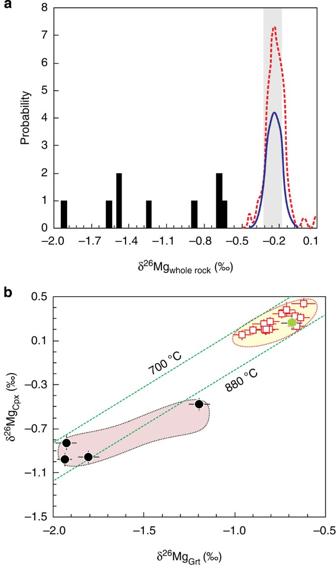Figure 1: Magnesium isotopic compositions of carbonated and normal eclogites. (a) Histogram of whole-rock δ26Mg of carbonated eclogites. The grey band represents the ‘normal’ mantle value14; the red dashed and blue solid curves are kernel density estimates of δ26Mg values of the normal eclogites from Sulu orogen and the Neoproterozoic basaltic protoliths from South China Block30, respectively. δ26Mg values of carbonated eclogites, represented by the histogram, are significantly lighter than both normal eclogites and their protoliths; (b) δ26Mg values of garnet (δ26MgGrt) and pyroxene (δ26MgCpx) separates from the normal and carbonated eclogites. The green hexagon represents the mineral separates from a normal eclogite close to the UHPM marble in the Rongcheng area. The red squares are mineral separates from normal eclogites in Chinese Continental Scientific Drill (CCSD). The black circles represent the mineral separates from carbonated eclogites. Green dotted lines are the equilibrium garnet–pyroxene Mg isotope fractionation lines51. Magnesium isotopic data are fromSupplementary Tables 2–4. The primary mineral assemblage of the carbonated eclogite is garnet, clinopyroxene, quartz, plagioclase and amphibole, with accessory minerals of calcite, dolomite, pyrrhotite, chalcopyrite and rutile ( Supplementary Table 1 ). Garnet and pyroxene minerals in carbonated eclogites are enriched in Ca relative to those in normal eclogites because of the UHPM metasomatism by host marbles [27] . The marbles range from calcite-rich to dolomite-rich in composition, and consist mainly of calcite and dolomite with silicate mineral assemblage of plagioclase, quartz and other minor phases such as pyroxene, amphibole, olivine and talc. Calcite contains significant MgO up to 4.43 wt. %, and dolomite has MgO in the range of 16.57~21.84 wt. % (refs 28 , 29 ). Magnesium isotopes The δ 26 Mg values of normal eclogites vary from −0.440 to +0.092‰, with an average value of −0.224±0.048‰ ( n =26; Fig. 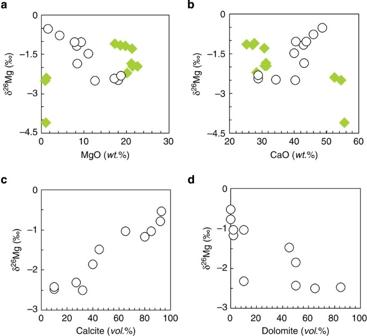Figure 2: Magnesium isotopic compositions of UHPM marbles and Sinian carbonates. (a) δ26Mg—MgO variations of UHPM marbles and Sinian carbonates; (b) δ26Mg—CaO variations of UHPM marbles and Sinian carbonates; (c) the variation of δ26Mg against calcite abundance in UHPM marbles; (d) the variation of δ26Mg against dolomite abundance in UHPM marbles. The white circles represent the UHPM marbles and the green diamonds represent the Sinian carbonates. Magnesium isotopic and major elemental data are fromSupplementary Table 3; mineral abundances are fromSupplementary Table 5. 1a and Supplementary Table 2 ), similar to that of their Neoproterozoic basaltic protoliths (δ 26 Mg=−0.196±0.044‰; Fig. 1a ) [30] . Garnets from these normal eclogites are systemically lighter than coexisting pyroxenes (Δ 26 Mg Cpx–Grt =δ 26 Mg Cpx −δ 26 Mg Grt =0.887–1.099‰), with δ 26 Mg ranging from −0.943 to −0.622‰ in garnets and from +0.151 to +0.438‰ in pyroxenes ( Fig. 1b and Supplementary Table 2 ). By contrast, carbonated eclogites are highly depleted in 26 Mg as compared with the normal eclogites, with δ 26 Mg varying from −1.928 to −0.648‰ ( Fig. 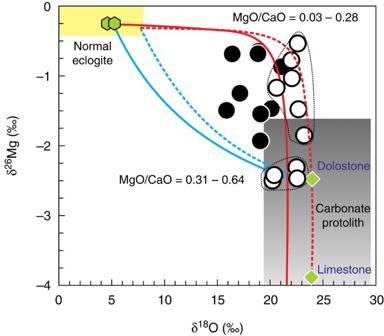Figure 3: Magnesium and O isotopic exchange between UHPM marbles and enclosed eclogites. The UHPM marbles and carbonated eclogites are represented by the white and black circles, respectively. Two end members of marble protoliths, limestone and dolostone are considered to have initial chemical compositions of Mg0.001Ca0.999CO3and Mg0.5Ca0.5CO3, respectively. Their O and Mg isotopic compositions are: δ18O=+24‰ and δ26Mg=−4.00‰ for limestone, and δ18O=+24‰ and δ26Mg=−2.50‰ for dolostone. The eclogites are assumed to have initial δ18O of +5.5‰, δ26Mg of −0.25‰ and MgO=8wt.%. The green hexagons represent two normal eclogites in gneisses close to the UHPM marble in the Rongcheng area. Equations that govern the isotopic exchange model are given inSupplementary Note 1. The red and blue curves represent the isotopic exchange of normal eclogites with limestone and with dolostone, respectively. The solid curves represent the Mg–O isotopic evolution of eclogites and the dashed curves represent the Mg–O isotopic evolution of marbles by isotopic exchange. The δ18O ranges of Sinian carbonates19and normal eclogites23are shown for comparison. Magnesium and O isotopic data are fromSupplementary Tables 2 and 3. 1a and Supplementary Table 3 ). These Mg isotopic ratios are the lightest known values in silicate rocks. The amphibolitic margin (11RC−2E) and eclogitic core (11RC−1) of an individual retrograded eclogite block (with diameter of ~30 cm) have δ 26 Mg of −0.648‰ and −0.684‰ ( Supplementary Table 3 ), respectively. Garnet and pyroxene separates from carbonated eclogites also have the lightest δ 26 Mg values ( Fig. 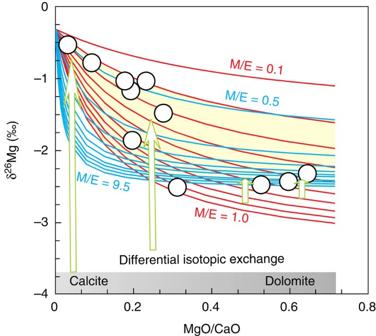Figure 4: Differential isotopic exchanges of eclogites with calcite-rich and dolomite-rich marbles. The eclogites are assumed to have initial δ26Mg of −0.25‰ and MgO=8wt.%. Equations that govern differential isotopic exchange model are given in theSupplementary Note 2. At a given weighted ratio of carbonate to eclogite (M/E) during isotopic exchange, marbles with different compositions (limestone versus dolostone) shift their δ26Mg in different degrees (shown by arrows). The red and blue curves assume that the initial δ26Mg of carbonates are −4.00‰ and −2.50‰, respectively. Different curves represent the isotopic exchange under different M/E ratios. The increment of M/E ratio is 0.1 for the red and 1.0 for the blue. Data are fromSupplementary Table 3. 1b and Supplementary Table 4 ), that is, from −1.937 to −1.191‰ in garnet and from −0.980 to −0.483‰ in pyroxene. Figure 1: Magnesium isotopic compositions of carbonated and normal eclogites. ( a ) Histogram of whole-rock δ 26 Mg of carbonated eclogites. The grey band represents the ‘normal’ mantle value [14] ; the red dashed and blue solid curves are kernel density estimates of δ 26 Mg values of the normal eclogites from Sulu orogen and the Neoproterozoic basaltic protoliths from South China Block [30] , respectively. δ 26 Mg values of carbonated eclogites, represented by the histogram, are significantly lighter than both normal eclogites and their protoliths; ( b ) δ 26 Mg values of garnet (δ 26 Mg Grt ) and pyroxene (δ 26 Mg Cpx ) separates from the normal and carbonated eclogites. The green hexagon represents the mineral separates from a normal eclogite close to the UHPM marble in the Rongcheng area. The red squares are mineral separates from normal eclogites in Chinese Continental Scientific Drill (CCSD). The black circles represent the mineral separates from carbonated eclogites. Green dotted lines are the equilibrium garnet–pyroxene Mg isotope fractionation lines [51] . Magnesium isotopic data are from Supplementary Tables 2–4 . Full size image Sinian carbonates comprise limestone (MgO/CaO=0.02) and dolostone (MgO/CaO=0.62~0.73), with δ 26 Mg varying from −4.101 to −2.396‰ in limestone and from −2.210 to −1.009‰ in dolostone ( Fig. 2a,b and Supplementary Table 3 ). The generally lighter δ 26 Mg in limestone than in dolostone is consistent with previous studies of normal sedimentary carbonates [16] , [17] , [18] . By contrast, δ 26 Mg values of the UHPM marbles vary from −2.508 to −0.531‰ and form a negative correlation with the dolomite abundance and a positive correlation with the calcite abundance ( Fig. 2c,d and Supplementary Table 3 ). Figure 2: Magnesium isotopic compositions of UHPM marbles and Sinian carbonates. ( a ) δ 26 Mg—MgO variations of UHPM marbles and Sinian carbonates; ( b ) δ 26 Mg—CaO variations of UHPM marbles and Sinian carbonates; ( c ) the variation of δ 26 Mg against calcite abundance in UHPM marbles; ( d ) the variation of δ 26 Mg against dolomite abundance in UHPM marbles. The white circles represent the UHPM marbles and the green diamonds represent the Sinian carbonates. Magnesium isotopic and major elemental data are from Supplementary Table 3 ; mineral abundances are from Supplementary Table 5 . Full size image Oxygen and other isotopes Two normal eclogites from Rongcheng have δ 18 O values of +5.65‰ and +3.96‰, respectively ( Supplementary Table 3 ). The δ 18 O of carbonated eclogites span a range of +15.9 to +21.1‰ ( Supplementary Table 3 ), which is consistent with previous studies of carbonated eclogites [31] . Neodymium isotope analyses of these carbonated eclogites yield initial ε Nd of −12.3 to −1.1 ( Supplementary Table 6 ), falling in the range of normal eclogites ( ε Nd =−16.7 to −0.1) [32] . The δ 18 O and δ 13 C of the UHPM marbles are in the ranges +20.3 to +23.3‰ and −2.01 to +4.77‰ ( Supplementary Table 3 ), respectively, similar to those of their protoliths [19] , [20] . Garnet and pyroxene from both normal and carbonated eclogites reach Mg isotopic equilibrium at peak metamorphic temperatures of 700~880 °C ( Fig. 1b ). The bulk carbonated eclogites and mineral separates have anomalously light δ 26 Mg and heavy δ 18 O values when compared with the normal eclogites and Neoproterozoic basaltic protoliths ( Fig. 1a,b ). Sedimentary limestones generally have lighter δ 26 Mg than dolostones [16] , [17] , [18] , whereas the UHPM marbles display the opposite trend, that is, isotopically heavy marbles have high CaO and low MgO contents ( Fig. 2a,b ). As such, the Mg–O isotopic signatures preserved in the carbonated eclogites and UHPM marbles do not reflect their protolith heterogeneity, rather they reflect carbonate–eclogite interactions during subduction including carbonate–eclogite mixing, metamorphic dehydration or rehydration, decarbonation and isotopic exchange. Carbonates are known to have extremely heavy δ 18 O and light δ 26 Mg values [16] , [17] , [18] , [19] , [20] ; thus, carbonate–eclogite mixing might explain the bulk Mg–O isotopic characteristics of carbonated eclogites. If we assume that eclogite lenses in marbles have initial δ 26 Mg and δ 18 O values similar to the normal eclogites, then a mixing calculation with carbonates indicates that ~60–90% contribution by carbonate is required to fit the bulk Mg–O isotopic compositions. However, the low CO 2 contents of carbonated eclogites (0.11–6.43 wt. %; Supplementary Table 3 ) imply that the calculated carbonate proportion is unrealistically high. In addition, carbonate–eclogite mixing predicts lighter δ 26 Mg values in those samples containing higher CO 2 contents, which is not seen in the carbonated eclogites ( Supplementary Fig. 2 ). Most importantly, garnet and pyroxene minerals in carbonated eclogites are equally enriched in 24 Mg and 18 O. This requires a chemical exchange rather than simple physical mixing between eclogite lenses and marbles. The Mg and O isotope fractionations between carbonated eclogites and their protoliths are far greater than predicted by closed-system metamorphic dehydration [30] , [33] . In addition, the δ 26 Mg of low MgO/CaO marbles are significantly heavier than the values of their pre-metamorphosed counterpart, Sinian limestones ( Fig. 2a,b ), which is opposite to the direction of isotope fractionation induced by metamorphic dehydration [34] . Thus, closed-system metamorphic dehydration is unlikely to account for the observed Mg–O isotopic variations in carbonated eclogites and UHPM marbles. Although the retrograded amphibolitic rim of an individual carbonated eclogite block has higher alkalies and CO 2 relative to the eclogitic core, they have similar Mg isotopic compositions ( Supplementary Table 3 ), ruling out the possibility of retrogression-induced Mg isotope fractionation. Metamorphic decarbonation involves the decomposition of a substantial amount of carbonate minerals by incorporating Mg and Ca oxides into the silicates and releasing CO 2 (ref. 35 ). This may explain the light δ 26 Mg and heavy δ 18 O of silicate minerals in carbonated eclogites. However, metamorphic decarbonation cannot significantly fractionate Mg isotopes, neither can it form the δ 26 Mg–CaO and δ 26 Mg–MgO correlations in UHMP marbles ( Fig. 2a,b ). Furthermore, previous studies have revealed that the subduction P–T trajectory of these carbonated eclogites and UHPM marbles does not intersect with experimentally determined carbonate-out boundaries ( Supplementary Fig. 3 ) [8] , suggesting limited decarbonation of these UHPM marbles. This is further supported by the similar O and C isotopic compositions between Sinian carbonates and UHPM marbles ( Supplementary Fig. 4 ), as large O and C isotope fractionations are expected during decarbonation [36] . The most likely process causing the Mg and O isotopic variations in carbonated eclogites and UHPM marbles is thus through fluid-mediated isotopic exchange. Previous studies revealed that Mg isotope fractionation between silicate and carbonate decreases dramatically from low temperatures (≥2‰ at T <300 °C) to high temperatures (0.05~0.08‰ at T =600~800 °C) [37] , [38] , [39] , [40] . Similar is true for O isotopes [33] . Therefore, extensive isotopic exchanges between marbles and eclogites are expected during prograde metamorphism to reduce their Mg and O isotopic differences. Assuming that sedimentary limestone and dolostone have heavy δ 18 O of +24‰ (ref. 19 ) but light δ 26 Mg around −4.00‰ and −2.50‰ (refs 16 , 17 , 18 ), respectively, and eclogite lenses in carbonates have initial Mg and O isotopic compositions similar to the normal eclogites (with average δ 18 O=+5.5‰ and δ 26 Mg=−0.25‰), the eclogites would become depleted in 26 Mg and enriched in 18 O after UHP isotopic exchange with the marbles ( Fig. 3 ). Magnesium isotopic exchange also elevated the δ 26 Mg values of UHPM marbles in various degrees ( Fig. 3 ). As limestone contains significantly lower Mg than dolostone, at a given weighted ratio between marble and eclogite the limestone is more susceptible than dolostone to Mg isotopic exchange with the eclogites ( Fig. 3 ). Consequently, the calcite-rich carbonates exhibit a large shift in δ 26 Mg towards heavier values, whereas the dolomite-rich carbonates tend to preserve their initial δ 26 Mg values ( Fig. 4 ). The negative co-variation of δ 26 Mg versus MgO/CaO for UHPM marbles ( Fig. 4 ) is therefore produced by the differential Mg isotopic exchange of compositionally varied carbonates with enclosed eclogite lenses. Figure 3: Magnesium and O isotopic exchange between UHPM marbles and enclosed eclogites. The UHPM marbles and carbonated eclogites are represented by the white and black circles, respectively. Two end members of marble protoliths, limestone and dolostone are considered to have initial chemical compositions of Mg 0.001 Ca 0.999 CO 3 and Mg 0.5 Ca 0.5 CO 3 , respectively. Their O and Mg isotopic compositions are: δ 18 O=+24‰ and δ 26 Mg=−4.00‰ for limestone, and δ 18 O=+24‰ and δ 26 Mg=−2.50‰ for dolostone. The eclogites are assumed to have initial δ 18 O of +5.5‰, δ 26 Mg of −0.25‰ and MgO=8 wt. %. The green hexagons represent two normal eclogites in gneisses close to the UHPM marble in the Rongcheng area. Equations that govern the isotopic exchange model are given in Supplementary Note 1 . The red and blue curves represent the isotopic exchange of normal eclogites with limestone and with dolostone, respectively. The solid curves represent the Mg–O isotopic evolution of eclogites and the dashed curves represent the Mg–O isotopic evolution of marbles by isotopic exchange. The δ 18 O ranges of Sinian carbonates [19] and normal eclogites [23] are shown for comparison. Magnesium and O isotopic data are from Supplementary Tables 2 and 3 . Full size image Figure 4: Differential isotopic exchanges of eclogites with calcite-rich and dolomite-rich marbles. The eclogites are assumed to have initial δ 26 Mg of −0.25‰ and MgO=8 wt. %. Equations that govern differential isotopic exchange model are given in the Supplementary Note 2 . At a given weighted ratio of carbonate to eclogite (M/E) during isotopic exchange, marbles with different compositions (limestone versus dolostone) shift their δ 26 Mg in different degrees (shown by arrows). The red and blue curves assume that the initial δ 26 Mg of carbonates are −4.00‰ and −2.50‰, respectively. Different curves represent the isotopic exchange under different M/E ratios. The increment of M/E ratio is 0.1 for the red and 1.0 for the blue. Data are from Supplementary Table 3 . Full size image Sedimentary carbonates are the main light-δ 26 Mg sink of Earth’s reservoirs [18] . Recycling of carbonates into the mantle has the potential to cause local mantle Mg isotope heterogeneity [41] . Knowledge of whether Mg isotopic compositions of sedimentary carbonates can be preserved during crustal subduction is fundamental to quantifying the amount of recycled carbonate in mantle sources using Mg isotopes. Our study suggests that calcite-rich carbonates are highly unlikely to retain their initial light δ 26 Mg but become isotopically heavier towards the value of silicates, whereas dolomite-rich carbonates are more capable of preserving their initial values. On the other hand, the carbonated silicates (for example, eclogites) gain light δ 26 Mg values that are significantly different from other normal eclogites and ambient mantle. These silicates may produce significant light-δ 26 Mg components in the mantle, as sampled by cratonic eclogites [42] and highly metasomatized peridotite xenoliths [43] . Magnesium isotopic analyses Magnesium isotopic analyses were carried out at the Isotope Laboratory of the University of Arkansas, Fayetteville, USA. Whole-rock powders of eclogites and carbonates, and the mineral separates were digested using Optima-grade mixed acid of HF-HNO 3 -HCl. After complete dissolution, dried residues from carbonate solutions were added 12 N HCl, and those from silicate solutions were taken up in 1 N HNO 3 for ion column chemistry. Detail column chemistry procedures have been reported elsewhere [44] , [45] . Chemical separation and purification of Mg were achieved by cation exchange chromatography with Bio-Rad AG50W-X8 resin in 1 N HNO 3 media. Additional chromatographic step was processed for the carbonate to further separate Mg from Ca by using Bio-Rad 200–400 mesh AG50W-X12 resin in 12 N HCl media. The same column procedure was performed twice in order to obtain the pure Mg recovery. The pure Mg solutions of silicate and carbonate were then dried down and re-dissolved in 3% HNO 3 ready for mass spectrometry. The Mg isotopic compositions were analysed by the sample-standard bracketing method using a Nu Plasma MC-ICPMS at low-resolution mode [46] . Each batch of sample analysis contains at least one well-characterized standard. Sample solution was repeated on ratio measurements for more than four times within a session. The long-term precision is better than ±0.07‰ (2 s.d.) for the 26 Mg/ 24 Mg ratio. Magnesium isotopic results are reported in the conventional δ notation in per mil relative to DSM-3, δ 26 Mg=[( 26 Mg/ 24 Mg) sample /( 26 Mg/ 24 Mg) DSM-3 −1] × 1,000. Oxygen–carbon and neodymium isotopic analyses Oxygen and carbon isotopic analyses were conducted at the CAS Key Laboratory of Crust-mantle Materials and Environments in the University of Science and Technology of China, Hefei. Oxygen isotopes of eclogites were measured by the laser fluorination technique. The O 2 was extracted by a CO 2 laser and transferred to a Finigan Delta+mass spectrometer for the measurement of 18 O/ 16 O and 17 O/ 16 O ratios. The O and C isotopes of carbonates were analysed by the GasBench II technique in the continuous flow mode and the extracted CO 2 gases were measured on a Finnigan MAT253 mass spectrometer. Detail procedures are described previously [47] . The O and C isotopic results are reported in the δ notation in per mil relative to Vienna Standard Mean Ocean Water and Vienna Peedee Belemnite, respectively. Samarium-Nd isotopic analyses were performed using an IsoProbe-T thermal ionization mass spectrometer at the State Key Laboratory of Lithospheric Evolution, Institute of Geology and Geophysics, Chinese Academy of Sciences. Samarium isotopes were measured using single Ta filament. Neodymium isotopes were determined using single tungsten filament with TaF 5 as an ionization activator. Detail column chemistry and mass spectrometer operation condition have been described previously [48] . 143 Nd/ 144 Nd ratios were corrected for mass fractionation using 146 Nd/ 144 Nd=0.7219. During the period of data collection, the measured value for the JNdi-Nd standard was 0.512117±10 (2 s.d.). Whole-rock chemistry and mineral abundances Major elements (except FeO, H 2 O + and CO 2 ) were analysed at the Hebei Institute of Regional Geology and Mineral Resources, China, by wavelength dispersive X-Ray fluorescence spectrometry [49] . The analytical uncertainties are better than 1%. The FeO contents of the samples were determined by conventional wet chemical method [50] . After the quantitative oxidation of Fe 2+ to Fe 3+ , the ferrous iron is regenerated by back-titration with ammonium ferrous sulfate. Then, the original Fe 2+ content can be calculated. H 2 O + and CO 2 were determined by gravimetric methods and potentiometry, respectively. The relative abundances of carbonate minerals were determined by X-ray diffraction using a Rigaku Smart lab (9 kW) at the China University of Geosciences, Beijing. The X-ray source was a Cu anode operated at 45 kV and 200 mA using CuKα 1 radiation equipped with a diffracted beam graphite monochromator. How to cite this article : Wang, S.-J. et al. Tracing carbonate–silicate interaction during subduction using magnesium and oxygen isotopes. Nat. Commun. 5:5328 doi: 10.1038/ncomms6328 (2014).